Measurement of cochlear power gain in the sensitive gerbil ear The extraordinary sensitivity of the mammalian ear is commonly attributed to the cochlear amplifier, a cellular process thought to locally boost responses of the cochlear partition to soft sounds. However, cochlear power gain has not been measured directly. Here we use a scanning laser interferometer to determine the volume displacement and volume velocity of the cochlear partition by measuring its transverse vibration along and across the partition. We show the transverse displacement at the peak-response location can be >1,000 times greater than the displacement of the stapes, whereas the volume displacement of an area centred at this location is approximately tenfold greater than that of the stapes. Using the volume velocity and cochlear-fluid impedance, we discover that power at the peak-response area is >100-fold greater than that at the stapes. These results demonstrate experimentally that the cochlea amplifies soft sounds, offering insight into the mechanism responsible for the cochlear sensitivity. Excitation of auditory sensory hair cells within the inner ear requires a sequence of mechanical steps, which commence when external airborne sounds pass through the ear canal and vibrate the flexible eardrum. This vibration reaches the cochlea via the middle-ear ossicular chain, displacing cochlear fluid and consequently vibrating the cochlear partition ( Fig. 1a ). The cochlear partition includes the flexible acellular basilar membrane and the cellular organ of Corti, which houses the sensory hair cells. A travelling wave of excitation starts at the base of the cochlear partition and propagates towards the apex. As the wave travels along the basilar membrane, its magnitude increases and speed decreases. The wave reaches its maximal magnitude at the best-frequency location, then quickly dies away beyond that place ( Fig. 1b,c ) [1] . Hair cells at the best-frequency location encode time, frequency and magnitude information of sounds and send them to the brain. In living cochleae, the vibration at the best-frequency site saturates as stimulus level is increased and displays sharp tuning as frequency is modulated [2] , [3] , [4] , [5] , [6] , [7] . Cochlear high sensitivity, sharp tuning and nonlinearity have been attributed to the cochlear amplifier, an active process derived from outer hair cells that has been proposed to amplify the basilar membrane response to soft sounds [8] , [9] , [10] , [11] , [12] , [13] , [14] , [15] , [16] . 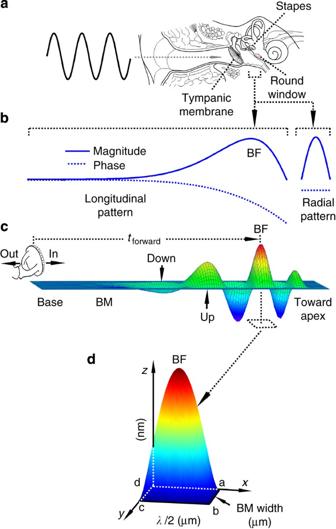Figure 1: Measurement of the volume displacement. (a) When a tone is presented to the ear, vibrations are measured along and across the basilar membrane through the round window and at the stapes footplates. (b) Magnitude and phase longitudinal and radial patterns of basilar membrane vibration. (c) The relationship between the stapes vibration and the cochlear forward travelling wave. (d) Volume displacement of basilar membrane vibration, measured as the volume bounded by the instantaneous waveform with a maximum displacement centred at the best-frequency location and the in-phase vibrating area on thexyplane (areaabcd). The length of this area is a half-wavelength and its width is approximately the basilar membrane width at the best-frequency location. BM, the basilar membrane; BF, best frequency;tforward, the forward delay;λ, the wavelength. Blue and red colours in panelscanddshow the low and high magnitude of the basilar membrane vibration, respectively. Figure 1: Measurement of the volume displacement. ( a ) When a tone is presented to the ear, vibrations are measured along and across the basilar membrane through the round window and at the stapes footplates. ( b ) Magnitude and phase longitudinal and radial patterns of basilar membrane vibration. ( c ) The relationship between the stapes vibration and the cochlear forward travelling wave. ( d ) Volume displacement of basilar membrane vibration, measured as the volume bounded by the instantaneous waveform with a maximum displacement centred at the best-frequency location and the in-phase vibrating area on the xy plane (area abcd ). The length of this area is a half-wavelength and its width is approximately the basilar membrane width at the best-frequency location. BM, the basilar membrane; BF, best frequency; t forward , the forward delay; λ , the wavelength. Blue and red colours in panels c and d show the low and high magnitude of the basilar membrane vibration, respectively. Full size image The gain of cochlear amplification is often estimated by comparing the ratio of basilar membrane-to-stapes vibration magnitude at low sound levels to that at high sound levels [2] (typically >100-fold or >40 dB). However, vibration magnitude at a single basilar membrane location does not provide information on the longitudinal and radial extent of the response nor indicates the energy of the vibration. Despite discovery of active force generation by outer hair cells through somatic motility and active bundle motion [17] , [18] and experimental studies of power flow in the cochlea [19] , [20] , [21] , [22] , the expected cochlear-amplifier power gain has yet to be demonstrated experimentally. By measuring the volume displacement and volume velocity, here we show that the cochlea, indeed, can generate energy and amplify basilar membrane vibration in response to soft sounds. We thus directly demonstrate power amplification in mammalian cochleae, which support the theory that the cochlear amplifier is responsible for the remarkable hearing sensitivity. Consistency of the data To quantify the energy gain of the basilar membrane vibration, we used a scanning laser interferometer to measure vibration not only at a single spot at the best-frequency location, but also along and across the basilar membrane. Because of the invasive surgery, extremely low reflectance of the cochlear partition [23] , vulnerability of cochlear sensitivity and time-consuming data collection, the productivity of the scanning measurements was low. Among 28 animals used in this study, 12 were excluded because of >8-dB hearing loss before data collection. No vibration data were collected from six animals because the poor transparency of the perilymph reduced the carrier signal and increased the noise floor. Incomplete longitudinal or radial data were collected from five cochleae due to deteriorating hearing during data acquisition. The sensitive scanning data presented here are thus from five cochleae, which had similar basilar membrane responses ( Fig. 2 ). 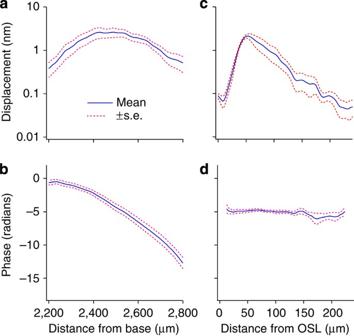Figure 2: Grouped magnitude and phase data of basilar membrane vibration. (a) The longitudinal magnitude pattern of the basilar membrane response to a 40-dB SPL 16-kHz tone, presented by means (blue solid line) and range of the standard error (red dotted lines) from five cochleae. (b) Corresponding longitudinal phase data. (c) Displacement magnitude as a function of the radial location. Standard errors near the osseous spiral lamina (OSL) are smaller than those in the region between 80 to 240 μm due to the relatively high reflectivity. (d) Corresponding radial phase data show little change across the basilar membrane. Figure 2: Grouped magnitude and phase data of basilar membrane vibration. ( a ) The longitudinal magnitude pattern of the basilar membrane response to a 40-dB SPL 16-kHz tone, presented by means (blue solid line) and range of the standard error (red dotted lines) from five cochleae. ( b ) Corresponding longitudinal phase data. ( c ) Displacement magnitude as a function of the radial location. Standard errors near the osseous spiral lamina (OSL) are smaller than those in the region between 80 to 240 μm due to the relatively high reflectivity. ( d ) Corresponding radial phase data show little change across the basilar membrane. 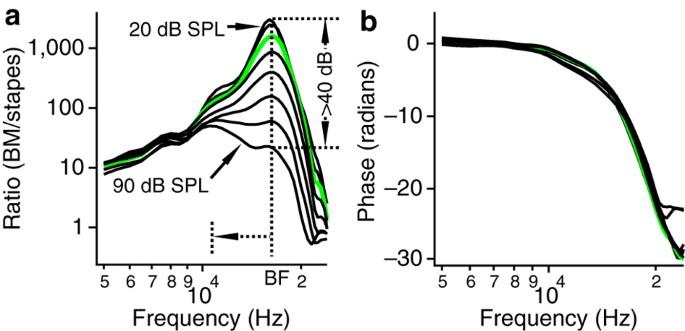Figure 3: Single-point basilar membrane vibration. The magnitude and phase of the basilar membrane vibration were measured at a single longitudinal location as a function of frequency. The ratio of basilar membrane-to-stapes vibration magnitude (BM/stapes) and phase difference between the stapes and basilar membrane are presented inaandb. (a) At 20–60 dB SPL, the magnitude increases with frequency and reaches the maximum at∼16 kHz. The magnitude and sharpness of the peak decreased with the sound level and the peak shifted to low frequencies from∼16 to∼11 kHz (horizontal dotted arrowed line). The magnitude at the peak frequency decreased >40 dB as the sound level increased from 20 to 90 dB SPL (indicated by vertical dotted arrowed lines). (b) The corresponding phase decreased progressively with frequency. The green curves show the responses at 40 dB SPL, the level used for quantifying the volume displacement in five sensitive cochleae. Full size image Basilar membrane vibration at a single location A typical data set of the basilar membrane vibration measured at a single location ∼ 2,500 μm from the base is presented in Figure 3 . Magnitude transfer functions, the ratio of the basilar membrane-to-stapes vibration magnitude as a function of frequency, are plotted in Figure 3a . At low and intermediate sound levels (20–60 dB SPL, wherein 0 dB SPL is 20 μPa), the basilar membrane vibrated maximally near 16 kHz, that is, the best frequency of the measured location. At sound levels of 20–40 dB SPL, the basilar membrane vibration at the best frequency was >1,000-fold greater than the stapes vibration. As the stimulus level increased from 20 to 90 dB SPL, the ratio decreased by >40 dB, indicating a compressive nonlinear growth. As the sound level increased, the response peak at ∼ 16 kHz becomes broader and shifted towards low frequencies. The green curves in Figure 3 show the response at 40 dB SPL, the level used for quantifying the volume displacement in five sensitive cochleae. The corresponding phase decreased progressively with frequency ( Fig. 3b ). The data in Figure 3 demonstrate that the sensitive cochlear preparations used in this study showed the same high sensitivity, nonlinearity and sharp tuning as reported previously [2] . Figure 3: Single-point basilar membrane vibration. The magnitude and phase of the basilar membrane vibration were measured at a single longitudinal location as a function of frequency. The ratio of basilar membrane-to-stapes vibration magnitude (BM/stapes) and phase difference between the stapes and basilar membrane are presented in a and b . ( a ) At 20–60 dB SPL, the magnitude increases with frequency and reaches the maximum at ∼ 16 kHz. The magnitude and sharpness of the peak decreased with the sound level and the peak shifted to low frequencies from ∼ 16 to ∼ 11 kHz (horizontal dotted arrowed line). The magnitude at the peak frequency decreased >40 dB as the sound level increased from 20 to 90 dB SPL (indicated by vertical dotted arrowed lines). ( b ) The corresponding phase decreased progressively with frequency. The green curves show the responses at 40 dB SPL, the level used for quantifying the volume displacement in five sensitive cochleae. 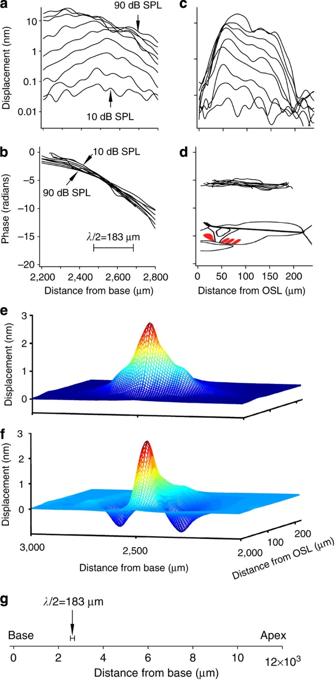Figure 4: Spatial patterns of basilar membrane vibration. Magnitude and phase of the basilar membrane vibration were measured as functions of the longitudinal and radial locations (a–d). The spatial pattern (e) and volume displacement (f) were calculated from the longitudinal and radial data. (a) At low sound levels from 10 to 40 dB SPL, the vibration increases with the distance from the cochlear base and forms a peak at∼2,500 μm. As the stimulus increased∼10,000-fold from 10 to 90 dB SPL, the response peak increased only∼100-fold, from∼0.1 to∼10 nm and shifted towards the base (left). (b) Phase decreased with longitudinal location. The phase slope became flatter at high sound levels. (c) Magnitude as a function of radial location, indicated by the distance from the osseous spiral lamina (OSL). The displacement magnitude varied significantly radially. (d) Phase show no significant change across the basilar membrane. Cartoon inset indicates the cross-section of the cochlear partition, with one inner hair cell (left) and three outer hair cells in red. (e) Magnitude spatial pattern of basilar membrane response to a 40-dB SPL 16-kHz tone. (f) Instantaneous waveform of the basilar membrane vibration. Blue and red colours ineandfshow the low and high magnitude of the basilar membrane vibration, respectively. (g) Spatial relationship of the quantified half wavelength and the basilar membrane length. Full size image Longitudinal patterns of basilar membrane vibration Scanning measurements of basilar membrane vibration at and around the best-frequency location are shown in Figure 4 . The magnitudes of cochlear partition vibrations measured at longitudinal locations ∼ 2,200 to ∼ 2,800 μm from the cochlear base are shown in Figure 4a . For a 16-kHz tone at intensities below 50 dB SPL, the best-frequency location was ∼ 2,500 μm from the base. As the stimulus magnitude increased 10,000-fold from 10 to 90 dB SPL, the displacement magnitude at the best-frequency location only increased about 100-fold, from ∼ 0.1 to ∼ 10 nm, indicating nonlinear compression of the response. At intensities below 50 dB SPL, the displacement-longitudinal location curves showed an approximately symmetrical peak centred at the best-frequency location. As the sound level increased, the response increased more in the basal direction than towards the apex, shifting the peak towards the base [24] , [25] . Figure 4: Spatial patterns of basilar membrane vibration. Magnitude and phase of the basilar membrane vibration were measured as functions of the longitudinal and radial locations ( a – d ). The spatial pattern ( e ) and volume displacement ( f ) were calculated from the longitudinal and radial data. ( a ) At low sound levels from 10 to 40 dB SPL, the vibration increases with the distance from the cochlear base and forms a peak at ∼ 2,500 μm. As the stimulus increased ∼ 10,000-fold from 10 to 90 dB SPL, the response peak increased only ∼ 100-fold, from ∼ 0.1 to ∼ 10 nm and shifted towards the base (left). ( b ) Phase decreased with longitudinal location. The phase slope became flatter at high sound levels. ( c ) Magnitude as a function of radial location, indicated by the distance from the osseous spiral lamina (OSL). The displacement magnitude varied significantly radially. ( d ) Phase show no significant change across the basilar membrane. Cartoon inset indicates the cross-section of the cochlear partition, with one inner hair cell (left) and three outer hair cells in red. ( e ) Magnitude spatial pattern of basilar membrane response to a 40-dB SPL 16-kHz tone. ( f ) Instantaneous waveform of the basilar membrane vibration. Blue and red colours in e and f show the low and high magnitude of the basilar membrane vibration, respectively. ( g ) Spatial relationship of the quantified half wavelength and the basilar membrane length. Full size image The phase of the basilar membrane response decreased with distance from the cochlear base ( Fig. 4b ), which indicated that waves travelled in the apical direction, that is, they formed a forward travelling wave [1] , [26] . At the basal side of the best-frequency location, the rate of phase decrease was small, indicating that the wave travelled rapidly through this region. As the observed location was moved through the best-frequency location towards the apex, the phase progressively decreased, indicating that the wave slowed. As sound level increased, the phase–longitudinal distance relation flattened modestly, indicating that wave travelled faster at high sound levels. Radial patterns of basilar membrane vibration Radial measurements of basilar membrane vibrations are shown in Figure 4c–d . As the sound level increased, the basilar membrane response increased in magnitude ( Fig. 4c ) but changed little in phase along the radial direction ( Fig. 4d ), consistent with previous reports [25] , [27] , [28] . The radial pattern of basilar membrane vibration magnitude was asymmetric across all sound levels ( Fig. 4c ); locations near the osseous spiral lamina vibrated at significantly higher magnitudes than those near the spiral ligament. At low levels (<30 dB SPL), basilar membrane vibration was mainly located over the region of ∼ 25–75 μm, where the hair cells are located. With increased sound level, the vibration spread both centrally and laterally. Spatial patterns of basilar membrane vibration To determine the volume displacement of the area of the cochlear partition centred at the best-frequency location (area abcd in Fig. 1d ), we measured the spatial patterns of basilar membrane vibration. Figure 4e shows the spatial envelope of the basilar membrane response to a 40-dB SPL 16-kHz tone; we calculated the instantaneous waveform ( Fig. 4f ) using magnitude and phase data (see Methods). The basilar membrane volume displacement is the volume bounded by the instantaneous waveform and the in-phase vibrating area centred at the best-frequency location ( Figs 1d and 4f ). The half-wavelength centred at the best-frequency location across sound levels was only 183 μm ( Fig. 4b ), which is ∼ 1.5% of the basilar membrane length ( Fig. 4g ). The size of this area suggests that fewer than 100 outer hair cells work in-phase for a 16-kHz tone at the best-frequency location. Volume displacement and power gain By measuring basilar membrane vibration at different sound pressure levels, we found that the volume displacement (solid line, Fig. 5a ) showed nonlinear compressive growth with stimulus level, whereas the growth of the stapes volume displacement (dotted line, Fig. 5a ) was linear. At 10 dB SPL, the cochlear volume displacement was approximately ten times greater than that of the stapes vibration; this ratio decreased as the sound level increased, and was unity at ∼ 80 dB SPL. 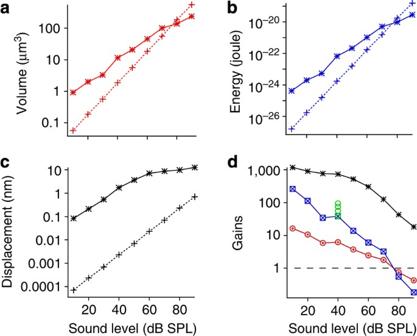Figure 5: Power gain of basilar membrane vibration. (a) Volume displacements of the basilar membrane (solid line) and stapes (dotted line) vibration as a function of the sound level. (b) Energy input and output functions of the basilar membrane (solid line) and stapes (dotted line) vibration. (c) Point displacements of the basilar membrane (solid line) and stapes (dotted line) vibration. (d) Energy (blue), volume- (red) and point- (black) displacement gains as a function of the sound level. Green circles show energy gains from five sensitive cochleae (mean=61, s.e.=11,n=5). Figure 5: Power gain of basilar membrane vibration. ( a ) Volume displacements of the basilar membrane (solid line) and stapes (dotted line) vibration as a function of the sound level. ( b ) Energy input and output functions of the basilar membrane (solid line) and stapes (dotted line) vibration. ( c ) Point displacements of the basilar membrane (solid line) and stapes (dotted line) vibration. ( d ) Energy (blue), volume- (red) and point- (black) displacement gains as a function of the sound level. Green circles show energy gains from five sensitive cochleae (mean=61, s.e.=11, n =5). Full size image The energy associated with basilar membrane vibration at the best-frequency location and near the stapes was calculated from the volume velocity and characteristic impedance of cochlear fluids (see Methods) and is displayed in Figure 5b . Although the shape of the energy input–output function of the basilar membrane at the best-frequency area (solid blue line, Fig. 5b ) was similar to that of the volume displacement (solid red line, Fig. 5a ), because energy depends on the square of the volume velocity, energy increased much more than the volume displacement when the sound level increased. As shown in Figure 5c , at low sound levels, the single-point basilar membrane vibration magnitude (solid line) was ∼ 1,000-fold greater than that of the stapes vibration (dotted line). Although the ratio decreased significantly at high sound levels, the basilar membrane vibration remained >10 times greater than the stapes vibration. The single-point data in Figure 5c is consistent with that in Figure 3a ; both show 30–40 dB compression. Ratios of the basilar membrane single-point displacement (black), volume displacement (red) or energy (blue) to the corresponding measures at the stapes (gains) are presented as a function of the sound level in Figure 5d . Green circles show energy gains from five sensitive cochleae (mean=61, s.e.=11, n =5). As the sound level increased from 10 to 90 dB SPL, single-point and volume displacement gains decreased by ∼ 30 dB, whereas the energy gain decreased as much as 60 dB; the energy gain of the cochlear partition vibration in response to low-level tones can be >100, yet dropped below 1 at high sound levels. Cochlear amplification was originally predicted by Gold [29] and was found to be possible by the ground-breaking discovery of otoacoustic emissions by Kemp [30] . In vitro experiments have indicated that electrical motility of outer hair cells [16] , [17] , [31] , [32] , [33] , [34] , [35] , [36] , [37] and active hair-bundle movement [16] , [17] , [31] , [32] , [33] , [34] , [35] , [36] , [37] can generate mechanical energy, whereas modelling studies [38] and accumulated experimental results [2] have supported the existence of cochlear amplification. Nevertheless, the expected cochlear power gain has not been demonstrated experimentally. Here, we measured the volume displacement and velocity of basilar membrane vibration, which, along with the cochlear-fluid impedance, allowed us to determine the associated energy. We found a power gain of ∼ 100 from cochlear base to best-frequency location, which provides the first direct experimental evidence of power amplification in the sensitive living cochlea. The principle for measuring the volume displacement or energy gain is the same as that for the conventional method for determining the single-point displacement gain [2] . In either case, the gain is quantified by the ratio of basilar membrane vibration magnitude at the best-frequency location to that of the stapes; the current and conventional methods are distinguished by different units, one of volume or energy and the other of length. Figure 1b,c shows the temporal and spatial relationships between the stapes and basilar membrane vibration. For a sinusoidal vibration, the volume displacement by the stapes footplates ( V s ) varies with time t and frequency f and is given by V s = V s+ • cos ( ωt ), where ω=2πf. V s+ is the absolute value of V s at t = nπ/ω ( n =0, 1, 2, ...), which is determined by multiplying the area of the stapes footplate with its point displacement [1] . As the vibration of the cochlear partition travels from the cochlear base to its best-frequency location, the magnitude may be reduced by damping or increased by the cochlear amplifier [8] , [9] , [11] , [12] , [13] , [14] , [16] , [39] . The volume displacement at the best-frequency location ( V bm ) is described by V bm = V bm+ • cos [ ω ( t + t forward )], where t forward is the forward delay of the basilar membrane vibration from the base to the best-frequency location ( Fig. 1b,c ). Similar to V s+ , V bm+ is the absolute value of V bm at t forward + nπ/ω ( n =0, 1, 2, ...), which is defined by the instantaneous waveform of basilar membrane vibration with the maximal volume displacement centred at the best-frequency location. The longitudinal extent of V bm is defined by the half-wavelength distance because the cochlear partition displaces in the same direction over this region, and the radial extent by the basilar membrane width (see Fig. 1d and Methods). This volume displacement differs from the net volume displacement over the basilar membrane length, which occurs simultaneously with the stapes vibration. The former is a measure of the travelling wave, whereas the later is related to the fast longitudinal wave [40] . At low sound levels, cochlear vibration is mostly restricted to the outer hair cell region ( Fig. 4c ) at the best-frequency area ( Fig. 4a ). Steep longitudinal phase slopes ( Fig. 4b ) indicate shorter wavelengths and smaller in-phase-vibration areas at low sound levels. For a given volume displacement or velocity, a smaller in-phase-vibration area results in a larger vibration in the transverse direction. Thus, in addition to level-dependent power amplification, the cochlea can increase the transverse vibration at the best-frequency location by focusing energy on the spatially restricted best-frequency region [41] . In turn, maximal transverse vibration optimally stimulates auditory sensory cells. Reflective of this focusing mechanism, the point-displacement gain (black line in Fig. 5d ) is about 100-fold greater than that of the volume displacement gain (red line in Fig. 5d ) at the low and intermediate sound levels. Because sharp cochlear tuning profits from a limited longitudinal extent of basilar membrane vibration [24] , the narrow longitudinal restriction of vibration contributes to cochlear sharp tuning. One may wonder whether the interferometer signal is from the basilar membrane or from deeper structures. Reflected light from a very reflective surface out of the focus might contribute to or even dominate the interferometer signal due to the large coherent length of lasers [42] , [43] , [44] . However, because of the difference in refraction index of the perilymph and the basilar membrane, incident light is reflected on the perilymph-basilar membrane interface in the current experiment. As a consequence of this reflection, the surface of the basilar membrane is visible through the microscope under the white light illumination. Because of the diffusion of the tissue, the structures on the scala-vestibuli side of the basilar membrane are not readily visible. Because the interferometer laser light is in the visible range of the spectrum, it too is subject to the same reflectivity as white light. Indeed, the carrier signal is optimized when the object beam is focused on the surface of the basilar membrane. Thus, the focal plane of the object beam was indicated by the optimal carrier signal and the sharpest image of the surface of the basilar membrane at the scala-tympani side. This was confirmed when we measured sound-induced vibration of the cochlear partition as a function of the transverse position using a low coherence interferometer with a visible light source. We found that the carrier signal was largest when the object beam was focused on the basilar membrane. In most classical cochlear mathematical models [26] , [39] , [40] , the cochlear travelling wave is presented by a series of independent sections along the longitudinal direction, and acoustic energy is transmitted dominantly through the cochlear fluid. According to these theories, the energy of the cochlear partition vibration at the best-frequency location can be quantified by measuring the power in the cochlear fluid surrounding the partition. Here, the fluid energy was quantified from the volume velocity and characteristic impendence of the cochlear fluid (see Methods). Because cochlear fluids may move radially and longitudinally, this method may underestimate the energy; our measured power gain of ∼ 100 should therefore be considered to be a lower bound. When the membrane potential of an outer hair cell changes as a result of sound-induced hair-bundle deflection, the cell body changes length and produces force due to a voltage-dependent conformational change in the membrane protein prestin [16] , [17] , [31] , [32] , [33] , [34] , [35] , [36] , [37] . Hair bundles of mammalian outer hair cells can also produce mechanical force [14] , [15] , [18] , [45] , [46] , [47] . In either case, outer hair cell-generated forces can enhance basilar membrane responses to soft sounds when the timing of force generation is appropriate [48] . The energy gain we observed in the living cochlea likely resulted from energy generated by somatic motility and/or active bundle motion of outer hair cells. Materials and general methods Twenty-eight young healthy Mongolian gerbils (40–80 g) were used in this study. Anaesthesia was induced by intraperitoneal injection of ketamine (30 mg kg −1 ) followed by intramuscular xylazine (5 mg kg −1 ) [24] . The animal use protocol was approved by the Oregon Health and Science University Institutional Animal Care and Use Committee. The method for measuring the basilar membrane vibration at a single longitudinal location was the same as previously [49] . Cochlear sensitivity was measured by recording the compound action potential and estimated by the nonlinear compression of basilar membrane responses. Scanning measurement of basilar membrane vibration The sensitivity of the laser interferometer was improved by increasing optical efficiency, which was achieved by removing the original collimating and focusing lenses and by precisely aligning different optical components [24] , [50] . The alignment result of each optical component was monitored using a compact laser power meter, and the optical sensitivity of the system was measured by the carrier signal levels when the object beam was focused on a low reflective ( ∼ 0.0001%) surface. The minimized noise floor of the instrument was achieved by maximizing the carrier signal level. For scanning measurements of the basilar membrane vibration, the transparency of the perilymph in the optical path significantly affected the carrier signal level and the noise floor. Blood cells suspended in the perilymph often prevented the interferometer from detecting the basilar membrane vibration. Great care was taken to minimize bleeding and to avoid blood cells entering the cochlea. Approximately 1 mm of basilar membrane in the first turn was exposed through the round window. The object beam of a scanning interferometer was focused on the basilar membrane through a glass coverslip and the perilymph. The scanning paths were determined by 10 to 20 reference points using a three-dimensional positioning system. The longitudinal scanning path was approximately underneath the second row of outer hair cells; the radial scanning path was at the best-frequency location. As the longitudinal position of the laser focus spot was changed at 5.0 μm s −1 , magnitudes and phases of the basilar membrane vibration velocity in response to a continuous best-frequency tone were collected at two samples per second, giving 0.4 sample per μm. The scanning rate along the radial direction was 2.0 μm s −1 , giving one sample per μm. The displacement magnitude ( D ) in nm and phase ( φ ) in radians at each location was calculated from the velocity magnitude ( V ) and phase ( θ ) according to D=V/2πf and φ=θ–π/2 , where f is the stimulus frequency in Hz. Volume displacement measurement Because radial phase patterns were approximately constant over a half-wavelength region along the longitudinal direction, we quantified the volume displacement of the basilar membrane vibration ( V bm ) as follows. The measured magnitude-radial location function was normalized with the maximum magnitude as 1.0; the radial magnitude pattern at each longitudinal location was obtained by multiplying the normalized radial magnitude pattern by the measured displacement at the given longitudinal location. The surface plot consisting of all displacement values over the in phase vibrating area shows the vibration magnitude in the space ( Fig. 4e ). The phase value at each location inside the in-phase vibrating area was obtained from the longitudinal and radial phase. To calculate the amplitude of the maximum volume displacement of the basilar membrane V bm+ , the phase value at the best-frequency location was shifted to nπ ( n =0, 1, 2...) by adding a constant to all phase values over the in-phase vibrating area. The instantaneous waveform ( Fig. 4f ) consists of the real value ( R ) at each location, which was derived from magnitude ( M p ) and phase ( φ p ) using R = M p * cos ( φ p ). V bm+ + was quantified by integrating R over the in-phase vibration area, which was defined by the basilar membrane width in the radial direction and a half-wavelength distance in the longitudinal direction (area abcd in Fig. 1d ). V s+ , the amplitude of the volume displacement of the stapes vibration was obtained from the product of D ps , the single-point displacement amplitude and A s , the area of the stapes footplate. D ps was taken approximately from the centre of the stapes footplate. Although complex stapes vibration has been reported [51] , our pilot experiments showed that vibrations from four distributed locations on the stapes footplate were in phase and that their mean was very close to the measured single-point displacement from the centre. In addition, the single-point vibration of the stapes has been commonly used for calculating the basilar membrane vibration transfer function [2] . To quantify A s , the stapes were collected and mounted using bone wax, with the perilymphatic surface of the stapes footplate in an approximately horizontal plane. The image of the stapes footplate was captured using a digital camera through a stereomicroscope. The edge of the stapes footplate was detected and A s was calculated by multiplying the number of pixels of stapes footplate image with the area of each pixel. The volume displacement gain of the basilar membrane vibration ( G vol ) was obtained according to G vol = V bm+ / V s+ at different intensities. The displacement gain measured from a single location ( G p ) was calculated using G p = D pbm / D ps , where D pbm and D ps are displacements at the best-frequency location and at the stapes. Measurement of energy and energy gain Despite a recent study [52] , most classical cochlear mathematical models [26] , [39] , [40] present the cochlear travelling wave using a series of independent sections along the longitudinal direction, and neglect longitudinal coupling. According to these theories, the relevant energy of the cochlear partition vibration can be quantified by measuring power in the cochlear fluid surrounding the partition. As energy in fluid can be quantified based on the volume velocity and fluid characteristic impedance [53] , the sound energy passing through the in-phase vibrating area centred at the best-frequency site in 1 s ( I bf ) was quantified according to the equation I bf = (V bfV ) 2 ρ c , where V bfV is the volume velocity measured centred at the best-frequency location ( V bfV =2 π f V bm+ , where f is frequency and V bm+ is the volume displacement), ρ is the density of the cochlear fluid ( ρ ≈1,000 kg m −3 ) and c is the speed of sound in water ( c ≈ 1,500 m s −1 ). Similarly, the energy in the cochlear fluid near the stapes ( I s ) was quantified according to equation I s = (V sV ) 2 ρ c , where V sV is the volume velocity of the stapes vibration ( V sV =2πf V s+ , where f is frequency and V s+ is volume displacement of the stapes vibration. The energy gain ( G e ) was obtained from equation G e = I bf / I s . According to the above relationship between energy and volume displacement, G e = G vol 2 , where G vol is the volume displacement gain. How to cite this article: Ren, T. et al . Measurement of cochlear power gain in the sensitive gerbil ear. Nat. Commun. 2:216 doi: 10.1038/ncomms1226 (2011).